Clustering of CARMA1 through SH3–GUK domain interactions is required for its activation of NF-κB signalling CARMA1-mediated NF-κB activation controls lymphocyte activation through antigen receptors and survival of some malignant lymphomas. CARMA1 clusters are formed on physiological receptor-mediated activation or by its oncogenic mutation in activated B-cell-diffuse large B-cell lymphomas (ABC-DLBCLs) with constitutive NF-κB activation. However, regulatory mechanisms and relevance of CARMA1 clusters in the NF-κB pathway are unclear. Here we show that SH3 and GUK domain interactions of CARMA1 link CARMA1 clustering to signal activation. SH3 and GUK domains of CARMA1 interact by either intra- or intermolecular mechanisms, which are required for activation-induced assembly of CARMA1. Disruption of these interactions abolishes the formation of CARMA1 microclusters at the immunological synapse, CARMA-regulated signal activation following antigen receptor stimulation as well as spontaneous CARMA1 clustering and NF-κB activation by the oncogenic CARMA1 mutation in ABC-DLBCLs. Thus, the SH3–GUK interactions that regulate CARMA1 cluster formations are promising therapeutic targets for ABC-DLBCLs. Nuclear factor κB (NF-κB) controls the activation and survival of lymphocytes. B-cell lymphoma 10 (BCL10) and mucosa-associated lymphoid tissue lymphoma translocation gene 1 (MALT1) form a complex essential for NF-κB activation signalling through immunoreceptor tyrosine-based activation motif-coupled receptors, G-protein-coupled receptors and epidermal growth factor receptor [1] , [2] , [3] . CARMA1, also known as caspase recruitment domain 11 (CARD11), is a member of the CARD-containing membrane-associated guanylate kinase (MAGUK) family (CARD-MAGUKs) and contains an amino-terminal CARD, a coiled-coil (C-C) domain, and a MAGUK signature motif comprising a PDZ domain, a Src homology 3 (SH3) domain and a GUK domain in the COOH terminus. CARMA1 forms a signalling complex with the BCL10-MALT1 through CARD–CARD interaction with BCL10, referred to as the lymphoid-CARMA1-BCL10-MALT1 (L-CBM) complex, following triggering through lymphocyte antigen receptors [1] . Genetic studies using gene-deficient mice and cell lines demonstrated that the L-CBM complex is essential for activation of the I-κB kinase (IKK) complex and the MAPK c-Jun N-terminal kinase (JNK) through antigen receptors and controls proliferation, survival and effector functions of lymphocytes [1] . CARMA1 functions as a molecular scaffold to organize a large signalling complex, including BCL10-MALT1, PKC, caspase 8, TRAF6, CK1α, Tak1, HPK1, PDK1, ADAP, CNS, A20 and IKK complex, to activate and modulate NF-κB signalling [4] . MAGUKs are modular scaffolds that regulate the formation and function of signalling complexes at cell–cell junctions [5] . All MAGUK proteins comprise one to three PDZ domains, an SH3 domain and a GUK domain that lacks catalytic activities but which acts as a protein interaction domain. Previous studies have suggested that organization of the protein complex by MAGUKs occurs through allosteric regulation of intra- and intermolecular interactions via the SH3 and GUK domains [6] , [7] , [8] , [9] , [10] , [11] , [12] . The importance of the SH3–GUK domain interaction for MAGUK function was demonstrated by genetic studies in invertebrates that identified numerous loss-of-function mutations in the SH3 and GUK domains of disc large (dlg) in Drosophila [13] and lin-2 in Caenorhabditis elegans [14] , all of which could disrupt SH3–GUK interactions [6] . However, it is unknown whether such mechanisms regulate CARMA1 function. We previously identified that CARMA1 accumulates and forms microclusters (MCs) with an annular appearance in the T-cell receptor (TCR)-CD3 lo region at the central supramolecular activation cluster (cSMAC) of the immunological synapse (IS) by a CD28-dependent co-stimulatory mechanism [15] , [16] . However, the molecular mechanisms regulating the cluster formation are not fully understood. In addition, it remains unclear whether the formation of CARMA1 clusters at the IS is physiologically relevant in the NF-κB activation pathway during antigen receptor signalling. Genetic evidence has established a pathogenic role for NF-κB signalling in tumours [17] . The L-CBM pathway is pathologically altered in several lymphoma subtypes [4] . Diffuse large B-cell lymphoma (DLBCL) is the most prevalent type of non-Hodgkin’s lymphoma, comprising 40% of cases [18] . Among the subtypes of DLBCLs, the least curable, aggressive, activated B-cell-like (ABC) subtype, but not the germinal centre B-cell-like (GCB) subtype, relies on constitutive NF-κB signalling. A loss-of-function RNA interference screen for genes required for survival of DLBCL revealed toxicity of short hairpin RNAs targeting CARMA1, MALT1 and BCL10 in ABC but not in GCB DLBCL cell lines [19] . In addition, ABC-DLBCL cell treatment with a MALT1 protease inhibitor reduced NF-κB activity resulting in death and growth retardation of ABC-DLBCL cells [20] , [21] . Oncogenic missense mutations of the CARD11 gene within exons encoding the C-C domain were observed in ABC-DLBCLs [19] . These missense CARD11 mutations resulted in a large aggregate formation of mutant CARMA1 proteins in the cytoplasm, and correlated with its ability to spontaneously activate the NF-κB pathway [22] . The oncogenic forms of CARMA1 are more potent than wild-type (WT) CARMA1 for inducing proteolytic activity of MALT1 (ref. 21 ). These observations indicated that dysregulation of CARMA1 clustering by oncogenic mutations might cause lymphomagenesis and malignancy by aberrant NF-κB activation. Thus, selective interference with L-CBM signalling is a promising strategy for ABC-DLBCL treatment and the suppression of CARMA1 cluster formation might be a therapeutic target. In this study, we demonstrate that the SH3 and GUK domains of CARMA1 can interact by either intra- or intermolecular mechanisms similar to previously reported MAGUKs. Lines of mutations that disrupt SH3–GUK interactions resulted in impaired NF-κB activation following antigen receptor stimulation. We identified that a previously reported fortuitous loss-of-function CARMA1 mutation in the SH3 domain, L815P [23] (in this manuscript, amino-acid (aa) numbering of human and mouse CARMA1 is according to NCBI Reference Sequence NP_115791.3 and NP_780571.2, respectively), disrupts SH3–GUK interactions. Mice bearing a L815P knock-in mutation showed defective development and activation of lymphocytes similar to those observed in CARMA1-null mice. Disruption of SH3–GUK interactions abolished the ability of CARMA1 to form MCs at the IS and aberrant large cluster formation as well as constitutive signal activation for NF-κB by the oncogenic CARMA1 mutant. Thus, SH3–GUK interactions are essential for both physiological and oncogenic cluster formation by CARMA1, and thereby control CARMA1-mediated signal activation in lymphocytes. We propose that SH3–GUK interactions might be novel therapeutic targets for ABC-DLBCLs. Self-interaction of CARMA1 through SH3 and GUK domains The molecular functions of the MAGUK region of CARMA1 remain obscure. To better understand signal regulation by CARMA1, we performed yeast two-hybrid screens to identify novel proteins that bind to the MAGUK region of CARMA1 using a mouse spleen complementary DNA library as the prey. We used two regions as baits: bait 1, a region between the 902 and 1154 aa sequence that contains the GUK domain, and bait 2, a region between the 648 and 901 aa sequence that contains the PDZ and SH3 domains ( Supplementary Fig. 1a ). We screened 4.0 × 10 7 colonies for bait 1 and 3.4 × 10 7 colonies for bait 2, and identified seven positive clones that interacted with bait 1, but none that interacted with bait 2. Sequence analysis revealed that all seven positive clones encoded an identical cDNA region from 407 to 860 aa of CARMA1, suggesting that CARMA1 self-associates through the GUK domain. To identify a specific region that interacted with the GUK domain, N-terminal and carboxy-terminal deletion constructs of the positive prey clone ( Supplementary Fig. 1b ) were co-transfected into HEK293 cells with the bait 1 construct and tested for interaction by co-immunoprecipitation assay ( Supplementary Fig. 1c ). We found that deletion of the SH3 domain completely abolished the interaction, indicating that the SH3 and GUK domains of CARMA1 interact. This interaction appears to be direct without bridging proteins as recombinant SH3 and GUK proteins were co-immunoprecipitated in vitro ( Supplementary Fig. 1d ). SH3–GUK modules of CARMA1 and PSD-95 have similar topology Interactions between SH3 and GUK domains have been reported in several other MAGUK family proteins [6] , [7] , [8] , [9] , [10] , [11] , especially in PSD-95, where the characteristics and structural requirements of the interaction have been investigated by biochemical and crystallographic studies [6] , [24] , [25] . Therefore, we compared the structure of the SH3–GUK module of CARMA1 with that of PSD-95. CARMA1 and PSD-95 exhibited 30% aa identity and 45% similarity in the SH3 domains, and 31% aa identity and 47% similarity in the GUK domains ( Supplementary Fig. 2a ). Notably, aa residues thought to be involved in the intermolecular SH3–GUK interaction of PSD-95 in a crystallographic study [24] were mostly conserved in CARMA1. In addition, the GUK domain lacked the canonical PxxP motifs recognized by typical SH3 domains and the SH3 domain lacked the conserved tyrosine residue, which is a crucial element for the recognition interface of PxxP-containing peptides [26] . This indicated that the SH3 and GUK domains of CARMA1 may not interact in a typical manner. Next we constructed a three-dimensional (3D) structure of the CARMA1 SH3–GUK module by homology modelling using the X-ray crystallographic structure of the rat PSD-95 SH3–GUK module (PDB ID: 1kjw) [25] . Since the 430–503 aa region containing the SH3 domain and αA helix and the 520–724 aa region containing the βE sheet and the GUK domain in PSD-95 were homologous with CARMA1, we developed a model of each comparable region in CARMA1. However, as the hinge region between the SH3 and GUK domains did not have significant sequence similarity, we did not include it. Modelling revealed that the secondary structures of the CARMA1 SH3–GUK module were similar to those of PSD-95 ( Supplementary Fig. 2a ). Importantly, a unique structural feature in the SH3–GUK module in PSD-95 seems to be conserved in CARMA1 in that, whereas the canonical SH3 fold has five continuous β strands (βA–βE) [26] , the SH3 folds in CARMA1 likely have six β strands (βA–βF) composed of discontinuous segments of sequence like PSD95 (refs 6 , 24 ), such that the hinge region separates βD and βE and the GUK domain is inserted between βE and βF ( Supplementary Fig. 2a,b ). This arrangement tethers the GUK domain to the SH3 βA–D fold through the βE/βF interface. Moreover, these structural features also seem to be conserved in the SH3–GUK modules in another CARD-MAGUK family, CARMA3, that regulates GPCR- and epidermal growth factor receptor-induced NF-κB activation in non-immune cells [2] , [3] ( Supplementary Fig. 3 ). SH3 and GUK can associate both in cis and trans fashion The crystal structure of the PSD-95 SH3–GUK module and biochemical studies suggest that the SH3–GUK interaction involves the assembly of a SH3 fold from two separate subdomains: β strands A–D of the SH3 fold and β strands E and F flanking the GUK fold ( Supplementary Fig. 2b ). In addition, the individual subdomains can assemble in an intra- or intermolecular manner, although the intermolecular form is favoured [6] , [25] . The presence of both βE and βF strands in the GUK fold is crucial to the interaction between the subdomains in PSD-95 (ref. 25 ). A predominance of the intramolecular interaction was observed in the CARMA1 SH3–GUK domain, as an isolated GUK domain of CARMA1 containing flanking βE and βF could associate only with a CARMA1 construct that contained a GUK domain truncation ( Fig. 1a,b ). A mutant of Dlg, dlg sw , bearing a COOH-terminal truncation following the GUK domain, comparable to a 13-aa truncation of PSD-95 containing the βF strand, disrupted the intramolecular SH3–GUK interaction both in Dlg and PSD-95 while leaving the SH3 and GUK domains intact [12] . The βF truncation of CARMA1 corresponding to the dlg sw mutation disrupted the intermolecular SH3–GUK interaction of CARMA1 ( Fig. 1c ), suggesting similarity in the biochemical interactions in CARMA1 and PSD-95. A different point mutation in Dlg, dlg m30 , that converts a conserved leucine in the SH3 domain to proline, corresponding to L460P in PSD-95, is sufficient to disrupt SH3–GUK interactions in PSD-95 (ref. 6 ). We found that the residue was conserved as a hydrophobic valine in the SH3 domain of CARMA1 ( Supplementary Fig. 2a ). Introduction of the same mutation to CARMA1 (V801P) disrupted the SH3–GUK interaction in CARMA1 ( Fig. 1d ; Supplementary Fig. 1d ). Crystallography demonstrated that Trp-471 in the SH3 domain of PSD-95 was involved in SH3–GUK interactions [24] . Although this residue is not conserved between PSD-95 and CARMA1, it has been reported that a point mutation at this position, L815P, in CARMA1 results in defective NF-κB activation induced by CD3/CD28 co-stimulation in Jurkat cells [23] . Surprisingly, we found that the integrity of this residue was required for SH3–GUK interactions of CARMA1 as the L815P mutation completely abrogated the interaction ( Fig. 1d ; Supplementary Fig. 1d ). 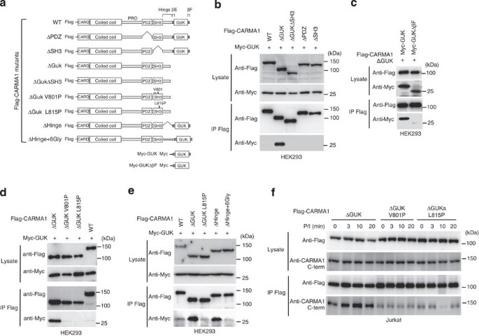Figure 1: Self-association of CARMA1 through SH3 and GUK domain interactions. (a) Schematic representation of the Flag-tagged WT and mutant constructs of CARMA1 and the Myc-tagged GUK and GUKΔβF constructs. (b–e) The Flag-tagged WT and mutant constructs of CARMA1 were co-transfected into HEK293T cells with Myc-tagged GUK (b–e) or GUKΔβF (c) constructs as indicated. The total cell lysates prepared from the transfected cells were immunoprecipitated with anti-Flag and subjected to immunoblot with anti-Myc. (f) Activation-induced intermolecular SH3–GUK domain interactions. Jurkat cells stably transduced with Flag-tagged CARMA1ΔGUK, CARMA1ΔGUKV801P or CARMA1ΔGUKL815P were stimulated with PMA (10 ng ml−1) plus calcium ionophore (1 μM) for the indicated times. Cell lysates were immunoprecipitated with anti-Flag and subjected to immunoblot with anti-CARMA1 that detects the COOH-terminal oligopeptides of endogenous CARMA1, but not the transduced CARMA1 mutants as they lack the COOH-terminal epitope sequence. Figure 1: Self-association of CARMA1 through SH3 and GUK domain interactions. ( a ) Schematic representation of the Flag-tagged WT and mutant constructs of CARMA1 and the Myc-tagged GUK and GUKΔβF constructs. ( b – e ) The Flag-tagged WT and mutant constructs of CARMA1 were co-transfected into HEK293T cells with Myc-tagged GUK ( b – e ) or GUKΔβF ( c ) constructs as indicated. The total cell lysates prepared from the transfected cells were immunoprecipitated with anti-Flag and subjected to immunoblot with anti-Myc. ( f ) Activation-induced intermolecular SH3–GUK domain interactions. Jurkat cells stably transduced with Flag-tagged CARMA1ΔGUK, CARMA1ΔGUKV801P or CARMA1ΔGUKL815P were stimulated with PMA (10 ng ml −1 ) plus calcium ionophore (1 μM) for the indicated times. Cell lysates were immunoprecipitated with anti-Flag and subjected to immunoblot with anti-CARMA1 that detects the COOH-terminal oligopeptides of endogenous CARMA1, but not the transduced CARMA1 mutants as they lack the COOH-terminal epitope sequence. Full size image The unusual SH3 fold allowing the domain–domain interaction of PSD-95 relies on the flexibility of the hinge region linking the two interacting subdomains [25] . The hinge region has been suggested to play an important role in determining the preference for inter- versus intramolecular assembly. Artificially reducing the flexibility of the hinge prevented intramolecular SH3–GUK interactions in PSD-95, and led to an intermolecular interaction through β strand swapping to complete the SH3 fold [25] . This result suggested an elegant model for a ligand-regulated oligomerization mechanism of PSD-95. Thus, we tested whether such regulation could be applied to CARMA1. Loss of flexibility by deleting the hinge region of CARMA1 (ΔHinge) promoted interactions between the SH3 domain and the GUK subdomain in neighbouring molecules, whereas replacement of the hinge with a flexible linker consisting of six glycines (ΔHinge+6Gly) inhibited the intermolecular interaction ( Fig. 1e ). These results indicated that the SH3–GUK fold of CARMA1 assembles preferentially to the intramolecular form, but also has a potential to exist between subdomains in the intermolecular form probably via 3D domain swapping ( Supplementary Fig. 4a ), as previously proposed in PSD-95 (ref. 25 ). Signal-induced CARMA1 assembly requires SH3–GUK interactions Previous reports have suggested that L-CBM proteins form oligomer and large signalling complex on activation [22] , [27] , [28] , [29] , [30] , [31] . To examine whether the SH3–GUK interactions contribute to the activation-dependent assembly of CARMA1, we developed human leukaemia Jurkat T cells stably expressing Flag-tagged CARMA1ΔGUK. In this setting, the SH3 domain from Flag-CARMA1ΔGUK can interact with the GUK-containing subdomain from endogenous CARMA1 when the limitation of intermolecular SH3–GUK interactions is released. In non-stimulated cells, an association between transduced CARMA1 and endogenous CARMA1 was present at very low levels. However, following cell stimulation with phorbol 12-myristate 13-acetate (PMA) plus Ca 2+ ionophore (P/I), a direct activator of PKCs, the association was considerably increased over time and peaked at 10 min ( Fig. 1f ), indicating that T-cell activation enhances assembly of CARMA1. However, the increase in CARMA1 assembly was not detected in resting or activated Jurkat cells stably expressing Flag-CARMA1ΔGUK with the V801P or L815P mutation. These results indicate that the SH3 and GUK interactions play an important role in the assembly of CARMA1 and regulated its degree on activation. TCR-induced NF-κB activation requires SH3–GUK interactions To investigate the role for the SH3–GUK interactions in TCR signalling for NF-κB activation, we transfected expression plasmids encoding WT or mutants (ΔCARD, ΔPDZ, ΔSH3, ΔGUK, ΔβF, V801P or L815P) of CARMA1 with an NF-κB-dependent luciferase reporter into CARMA1-deficient Jurkat cells (JPM50.6; Fig. 2a,b ; Supplementary Fig. 5a ). As previously reported [32] , JPM50.6 cells demonstrated defective NF-κB activation induced by PMA-CD28 co-stimulation ( Fig. 2a ) or by conjugation with Staphylococcal enterotoxin E (SEE)-loaded Raji B cells ( Fig. 2b ), where Raji cells present superantigens to the TCR complex as well as provide co-stimulation to CD28 on JPM50.6 cells, while the CARMA1 deficiency did not influence NF-κB activation induced by tumor necrosis factors (TNF; Fig. 2c ). As the CARD domain is essential for complex formation with BCL10, expression of the ΔCARD mutant could not rescue the defects of NF-κB signalling in JPM50.6 cells, whereas expression of WT CARMA1 or ΔPDZ mutant fully rescued the defects. This indicated that the PDZ domain was dispensable for NF-κB signalling. However, lack of the SH3 or the GUK domain (ΔSH3 or ΔGUK) as well as mutations that specifically disrupt the SH3–GUK interaction (ΔβF, V801P or L815P) completely abrogated the ability of CARMA1 to rescue the defects ( Fig. 2a,b ). Similar results were obtained when JPM50.6 cells stably transduced with WT or mutant CARMA1 were stimulated with anti-CD3/CD28 or P/I ( Supplementary Fig. 6 ). In contrast, expression of these mutants did not influence TNF-induced NF-κB activation ( Fig. 2c ), indicating that there was no bystander effect on the common NF-κB signalling pathway by overexpression of these mutants. These results clearly demonstrated an essential role for the SH3–GUK interactions in NF-κB activation induced by TCR co-stimulation in Jurkat cells. 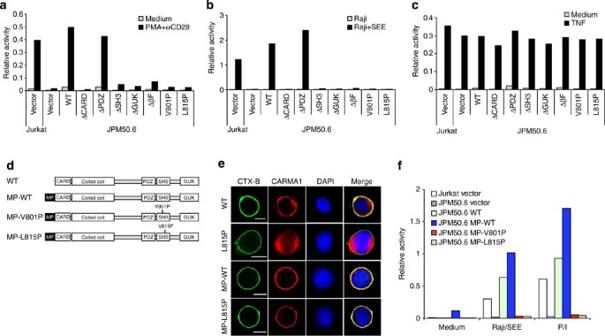Figure 2: Disruption of the SH3–GUK interactions abolishes TCR-co-stimulation-induced NF-κB activation in Jurkat T cells. (a–c,f) Jurkat or JPM50.6 cells were transfected with plasmids encoding an NF-κB luciferase reporter plasmid (Fireflyluciferase) together with expression plasmids encoding mock, WT CARMA1 or the mutant CARMA1 constructs indicated inFig. 1b,d. Twenty-four hours after transfection, transfected cells and Jurkat cells were left unstimulated or stimulated with PMA (10 ng ml−1) plus anti-CD28 (1 μg ml−1;a), PMA (10 ng ml−1) plus calcium ionophore (1 μM; P/I;f), non- or SEE (10 ng ml−1)-primed Raji cells (b,f) or TNF (10 ng ml−1;c) for 6 h. Cells were lysed and luciferase activity was determined. All samples were also transfected with constitutively expressedRenillaluciferase to normalize the transfection efficiency. (d) Schematic representation of WT and mutant CARMA1 constructs used ine,f. MP, myristoylation/palmitoylation motif of Lck. (e) JPM50.6 cells were stably reconstituted with WT CARMA1 or indicated CARMA1 mutants, labelled with DAPI (blue, for nuclear staining), FITC-conjugated cholera toxin β-subunit (CTX-B; green, for lipid raft staining) and rabbit anti-CARMA1 polyclonal antibody followed by TRITC-conjugated anti-rabbit IgG (red) and imaged by confocal microscopy. Scale bars, 5 μm. Figure 2: Disruption of the SH3–GUK interactions abolishes TCR-co-stimulation-induced NF-κB activation in Jurkat T cells. ( a – c , f ) Jurkat or JPM50.6 cells were transfected with plasmids encoding an NF-κB luciferase reporter plasmid ( Firefly luciferase) together with expression plasmids encoding mock, WT CARMA1 or the mutant CARMA1 constructs indicated in Fig. 1b,d . Twenty-four hours after transfection, transfected cells and Jurkat cells were left unstimulated or stimulated with PMA (10 ng ml −1 ) plus anti-CD28 (1 μg ml −1 ; a ), PMA (10 ng ml −1 ) plus calcium ionophore (1 μM; P/I; f ), non- or SEE (10 ng ml −1 )-primed Raji cells ( b , f ) or TNF (10 ng ml −1 ; c ) for 6 h. Cells were lysed and luciferase activity was determined. All samples were also transfected with constitutively expressed Renilla luciferase to normalize the transfection efficiency. ( d ) Schematic representation of WT and mutant CARMA1 constructs used in e , f . MP, myristoylation/palmitoylation motif of Lck. ( e ) JPM50.6 cells were stably reconstituted with WT CARMA1 or indicated CARMA1 mutants, labelled with DAPI (blue, for nuclear staining), FITC-conjugated cholera toxin β-subunit (CTX-B; green, for lipid raft staining) and rabbit anti-CARMA1 polyclonal antibody followed by TRITC-conjugated anti-rabbit IgG (red) and imaged by confocal microscopy. Scale bars, 5 μm. Full size image Studies suggest that recruitment of L-CBM molecules to plasma membrane lipid rafts regulate antigen receptor-induced NF-κB activation signals [1] , [33] . Although we observed that the L815P mutation abrogated the SH3–GUK interactions ( Fig. 1d ), Wang et al . [23] reported that the L815P mutation of CARMA1 resulted in defective membrane association of CARMA1. To determine which changes in the molecular properties is responsible for the signalling defects of this mutant, we transduced JPM50.6 cells with expression plasmids encoding WT, V801P or L815P of CARMA1 tagged at the NH 2 terminus with a myristoylation/palmitoylation (MP) motif derived from Lck tyrosine kinase [34] to target CARMA1 proteins to the plasma membrane lipid rafts ( Fig. 2d ; Supplementary Fig. 5b ). We observed that WT CARMA1 resided both in the cytoplasm and the plasma membrane, whereas the plasma membrane localization was lost in CARMA1 L815P ( Fig. 2e ) as reported by Wang et al . [23] In contrast, MP-tagged CARMA1 proteins were selectively localized to the plasma membrane irrespective of the L815P mutation. The forced membrane expression of WT CARMA1 substantially increased the basal and activation-induced NF-κB activity compared with native CARMA1 in the NF-κB reporter assay ( Fig. 4f ; Supplementary Fig. 5c ), consistent with the idea that CARMA1 function is regulated by the membrane recruitment [23] , [31] , [35] , [36] . However, the forced membrane expression could not rescue the disability of CARMA1 L815P to activate NF-κB signalling. The enhanced NF-κB activity by the membrane targeting of CARMA1 completely disappeared in the presence of the L815P or V801P mutations. Thus, the defective NF-κB activation governed by these point mutations is unlikely due to the defective membrane localization of CARMA1. Figure 4: SH3–GUK regulation is essential for B-cell physiology mediated by CARMA1. 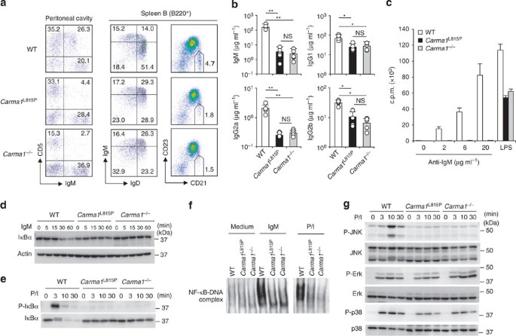Figure 4: SH3–GUK regulation is essential for B-cell physiology mediated by CARMA1. (a) Peritoneal IgM+CD5+B-1 cells and splenic follicular IgMloIgDhiB-2 and CD21hiCD23lomarginal zone B cells from 8-week-old WT,Carma1L815PandCarma1–/–mice were analysed by flow cytometry. Data are representative of four independent experiments. (b) Basal serum immunoglobulin levels in 8-week-old WT,Carma1L815PandCarma1–/–mice were analysed. Each circle represents an individual mouse; error bars indicate the s.d. *P<0.01 and **P<0.001 (Student’st-test). (c) Purified splenic B cells from WT,Carma1L815PandCarma1–/–mice were stimulated with the indicated amount of anti-IgM F(ab′)2or 1 μg ml−1of LPS for 48 h. Proliferation was measured by [3H]thymidine uptake. Data represent the mean±s.d. of triplicate cultures. (d–g) Purified splenic B cells from WT, Carma1L815PandCarma1–/–mice were stimulated with anti-IgM F(ab′)2(10 μg ml−1) or with PMA (10 ng ml−1) plus calcium ionophore (1 μM; P/I) for the indicated times. Cell lysates were analysed by immunoblotting of actin (d), total (d,e) and phosphorylated IκBα (e) and total and phosphorylated JNK, ERK and p38 (g). (f) The electrophoretic mobility shift assay. Nuclear extracts were prepared from purified WT,Carma1L815PandCarma1–/–splenic B cells stimulated for 8 h with anti-IgM F(ab′)2and P/I. Electromobility shift assays were performed using DIG-labelled oligonucleotide probes containing consensus NF-κB-binding sites. Results are representative of more than three independent experiments. ( a ) Peritoneal IgM + CD5 + B-1 cells and splenic follicular IgM lo IgD hi B-2 and CD21 hi CD23 lo marginal zone B cells from 8-week-old WT, Carma1 L815P and Carma1 –/– mice were analysed by flow cytometry. Data are representative of four independent experiments. ( b ) Basal serum immunoglobulin levels in 8-week-old WT, Carma1 L815P and Carma1 –/– mice were analysed. Each circle represents an individual mouse; error bars indicate the s.d. * P <0.01 and ** P <0.001 (Student’s t -test). ( c ) Purified splenic B cells from WT, Carma1 L815P and Carma1 –/– mice were stimulated with the indicated amount of anti-IgM F(ab′) 2 or 1 μg ml −1 of LPS for 48 h. Proliferation was measured by [ 3 H]thymidine uptake. Data represent the mean±s.d. of triplicate cultures. ( d – g ) Purified splenic B cells from WT, Carma1 L815P and Carma1 –/– mice were stimulated with anti-IgM F(ab′) 2 (10 μg ml −1 ) or with PMA (10 ng ml −1 ) plus calcium ionophore (1 μM; P/I) for the indicated times. Cell lysates were analysed by immunoblotting of actin ( d ), total ( d , e ) and phosphorylated IκBα ( e ) and total and phosphorylated JNK, ERK and p38 ( g ). ( f ) The electrophoretic mobility shift assay. Nuclear extracts were prepared from purified WT, Carma1 L815P and Carma1 –/– splenic B cells stimulated for 8 h with anti-IgM F(ab′) 2 and P/I. Electromobility shift assays were performed using DIG-labelled oligonucleotide probes containing consensus NF-κB-binding sites. Results are representative of more than three independent experiments. Full size image PDK1 and ADAP are important signalling mediators through TCRs for NF-κB activation and interact with the GUK domain and MAGUK region of CARMA1, respectively [35] , [36] . Co-immunoprecipitation studies revealed that V801P and L815P mutations did not affect the association of CARMA1 with these mediators ( Supplementary Fig. 4b,c ), indicating that defective NF-κB activation by these SH3 mutations is unlikely due to the defective interaction of CARMA1 with PDK1 or ADAP. SH3–GUK regulation controls T-cell development/activation To determine the physiological relevancy of the signalling regulation of CARMA1 by the SH3–GUK interactions, we generated knock-in mice harbouring an L815P mutation in CARMA1 ( Carma1 L815P ) ( Supplementary Fig. 7 ). The knock-in mutation in mice did not alter CARMA1 expression levels in peripheral lymphocytes irrespective of activation status ( Supplementary Fig. 8a ). Notably, the subcellular localization of mutant CARMA1 was not altered in primary T cells ( Supplementary Fig. 8b ), in contrast to that in Jurkat cells. Overall development of conventional CD4 + and CD8 + T cells in the thymus, lymph nodes and spleen was not impaired in Carma1 L815P mice ( Supplementary Fig. 9a,b ). However, Carma1 L815P mice had defects in the development of naturally occurring CD4 + CD8 – Foxp3 + regulatory T cells (nTregs) similar to Carma1 –/– mice, albeit to a slightly lesser extent ( Fig. 3a ). Lymph node T cells isolated from Carma1 L815P and Carma1 –/– mice showed markedly attenuated proliferation ( Fig. 3b ) and almost completely abolished interleukin (IL)-2 production ( Fig. 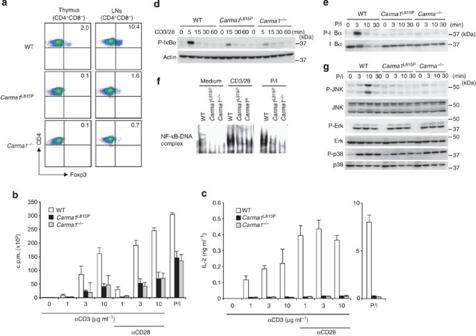3c ) following TCR, TCR/CD28 or P/I stimulation, indicating that the SH3–GUK interactions are essential for T-cell activation through the TCR downstream of PKC. Figure 3: SH3–GUK regulation is essential for T-cell physiology mediated by CARMA1. (a) CD4+CD8–FOXP3+naturally occurring regulatory T cells (nTreg) in the thymus (left) and inguinal lymph nodes (right) from 8-week-old WT,Carma1L815PandCarma1–/–mice were analysed by flow cytometry. Data are representative of four independent experiments. (b,c) Proliferation (b) and IL-2 production (c) of purified lymph node T cells from WT,Carma1L815PandCarma1–/–mice after stimulation with indicated amounts of plate-bound anti-CD3ε with or without 1 μg ml−1of plate-bound anti-CD28, or with PMA (10 ng ml−1) plus calcium ionophore (1 μM; P/I) for 48 h. Proliferation was measured by [3H]thymidine uptake. Data inb,crepresent the mean±s.d. of triplicate cultures. (d,e,g) Purified lymph node T cells from WT,Carma1L815PandCarma1–/–mice were treated with anti-CD3ε plus anti-CD28 (10 μg ml−1of each) followed by crosslinking with anti-hamster antibody (10 μg ml−1;d) or stimulated with P/I (e,g) for the indicated times. Cell lysates were analysed by immunoblotting for total (e) and phosphorylated IκBα (d,e) and for total and phosphorylated JNK, ERK and p38 (g). (f) The electrophoretic mobility shift assay. Nuclear extracts were prepared from purified WT,Carma1L815PorCarma1–/–lymph node T cells stimulated for 8 h with plate-bound anti-CD3ε plus anti-CD28 (10 μg ml−1of each) and P/I. Electromobility shift assays were performed using DIG-labelled oligonucleotide probes containing consensus NF-κB-binding sites. Results are representative of more than three independent experiments. Figure 3: SH3–GUK regulation is essential for T-cell physiology mediated by CARMA1. ( a ) CD4 + CD8 – FOXP3 + naturally occurring regulatory T cells (nTreg) in the thymus (left) and inguinal lymph nodes (right) from 8-week-old WT, Carma1 L815P and Carma1 –/– mice were analysed by flow cytometry. Data are representative of four independent experiments. ( b , c ) Proliferation ( b ) and IL-2 production ( c ) of purified lymph node T cells from WT, Carma1 L815P and Carma1 –/– mice after stimulation with indicated amounts of plate-bound anti-CD3ε with or without 1 μg ml −1 of plate-bound anti-CD28, or with PMA (10 ng ml −1 ) plus calcium ionophore (1 μM; P/I) for 48 h. Proliferation was measured by [ 3 H]thymidine uptake. Data in b , c represent the mean±s.d. of triplicate cultures. ( d , e , g ) Purified lymph node T cells from WT, Carma1 L815P and Carma1 –/– mice were treated with anti-CD3ε plus anti-CD28 (10 μg ml −1 of each) followed by crosslinking with anti-hamster antibody (10 μg ml −1 ; d ) or stimulated with P/I ( e , g ) for the indicated times. Cell lysates were analysed by immunoblotting for total ( e ) and phosphorylated IκBα ( d , e ) and for total and phosphorylated JNK, ERK and p38 ( g ). ( f ) The electrophoretic mobility shift assay. Nuclear extracts were prepared from purified WT, Carma1 L815P or Carma1 –/– lymph node T cells stimulated for 8 h with plate-bound anti-CD3ε plus anti-CD28 (10 μg ml −1 of each) and P/I. Electromobility shift assays were performed using DIG-labelled oligonucleotide probes containing consensus NF-κB-binding sites. Results are representative of more than three independent experiments. Full size image Next we analysed TCR-induced signal activation in Carma1 L815P T cells. Phosphorylation of IκBα was markedly impaired following TCR/CD28 stimulation ( Fig. 3d ) and completely abolished following P/I stimulation ( Fig. 3e ) in Carma1 L815P T cells similar to Carma1 –/– T cells. Consistently, the DNA-binding activity of NF-κB in the nuclei of Carma1 L815P T cells following TCR/CD28 or P/I stimulation was impaired similar to Carma1 –/– T cells ( Fig. 3f ; Supplementary Fig. 10 ). In addition, activation of JNK, but not ERK and p38, in Carma1 L815P T cells following P/I stimulation was markedly impaired similar to Carma1 –/– T cells ( Fig. 3g ). These results suggested that the SH3–GUK interactions are essential for CARMA1-mediated signal activation in primary T cells. SH3–GUK regulation controls B-cell development/activation Next we analysed B-cell development and activation in Carma1 L815P mice. As previously reported in Carma1 –/– mice [37] , [38] , Carma1 L815P mice showed reduced mature B220 + IgD hi IgM lo follicular and B220 + CD21 hi CD23 lo marginal zone B cells in the spleen compared with WT mice, and an almost complete absence of peritoneal IgM + CD5 + B-1 B cells in Carma1 L815P mice ( Fig. 4a ; Supplementary Fig. 9c ). In addition, Carma1 L815P mice showed markedly reduced serum IgM and IgG levels, similar to those in Carma1 –/– mice ( Fig. 4b ). Consistently, proliferative responses to anti-IgM were almost completely abrogated in Carma1 L815P splenic B cells, similar to that in Carma1 –/– B cells ( Fig. 4c ). In addition, proliferation of Carma1 L815P and Carma1 –/– B cells in response to lipopolysaccharide (LPS) was similarly partially attenuated [37] . Next we analysed B-cell receptor (BCR)-induced signal activation in Carma1 L815P B cells. Degradation of IκBα ( Fig. 4d,e ) and the DNA-binding activity of NF-κB in the nuclei ( Fig. 4f ) following BCR crosslinking or P/I stimulation was almost completely abolished in Carma1 L815P B cells similar to Carma1 –/– B cells. In addition, activation of JNK, but not ERK and p38, following P/I stimulation was almost completely abolished in Carma1 L815P as Carma1 –/– B cells ( Fig. 4g ). Thus, similar to T cells, the SH3–GUK interactions are essential for CARMA1-mediated signal activation in primary B cells. IS CARMA1 cluster formation depends on SH3–GUK interactions We previously demonstrated that CARMA1 and PKC-θ form MCs at the CD3 lo region of cSMAC in the IS, which is dependent on CD28 co-stimulation, suggesting that CD3 lo signalling cSMAC may function as a signallosome for NF-κB activation [15] , [16] . However, the physiological relevancy of CARMA1 MCs in NF-κB signalling is unknown. Thus, we explored the functional association of the SH3–GUK interactions with MC formation of CARMA1. CD4 + T cells from AND TCR transgenic (AND-Tg; specific for moth cytochrome c 88–103 (MCC88–133) on I-E k ) mice were retrovirally transduced with enhanced green fluorescent protein (EGFP)-tagged WT CARMA1 or mutant CARMA1 (V801P or L815P). Note that expression levels of transduced GFP-tagged CARMA1s were comparable to that of endogenous CARMA1 and were comparable between samples ( Supplementary Fig. 11a ). The transfected T cells were added onto a planar bilayer containing glycophosphatidylinositol (GPI)-anchored I-E k loaded with MCC88-133, ICAM-1-GPI and CD80-GPI, and movement of the EGFP-CARMA1 molecules was imaged. WT-, V801P- and L815P-mutant CARMA1 were uniformly distributed in the cytoplasm without forming visible clusters before attachment to the bilayer ( Fig. 5a ). As previously reported [16] , TCR-CD3 MCs were formed soon after T cells became attached (2 min) and at a later stage (30 min) translocated to the cSMAC. In contrast, CARMA1 MCs were induced at a later stage and accumulated at the TCR lo region surrounding the central TCR hi region within cSMACs in the annular structure ( Fig. 5a ). We observed that the CARMA1 MC formation was almost completely abrogated by V801P or L815P mutation ( Fig. 5a,b ). The same defect was observed for Carma1 L815P T cells in experiments using a specific antibody for CARMA1 ( Supplementary Fig. 12 ). These results suggested an indispensable role for the SH3–GUK domain interactions in CARMA1 MC formation, and further suggested the relevancy of the CARMA1 MCs at IS as signallosomes for NF-κB activation signalling. 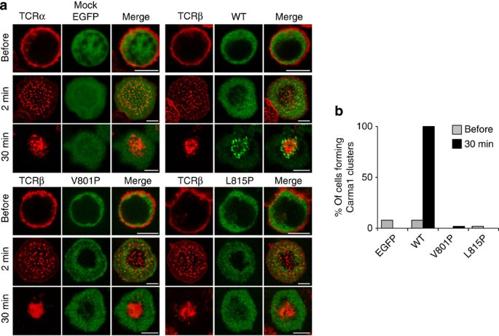Figure 5: The SH3–GUK interaction is essential for the formation of CARMA1 microclusters at the IS. (a) AND-Tg T cells expressing a mock-monomeric EGFP or WT, V801P or L815P CARMA1-mEGFP (green) were stained for TCRβ with DyLight 649-conjugated H57 F′ab (red), plated onto an MCC88-103-prepulsed planar bilayer containing I-Ek-, ICAM-1- and CD80-GPI and imaged by confocal microscopy at 2 and 30 min after contact. Images of cells before attachment to the bilayer were taken at the equatorial plane of the cells. The percentage of cells forming CARMA1 microclusters at 30 min after contact is shown inb(n=50). A representative of three independent experiments is shown. Scale bars, 5 μm. Figure 5: The SH3–GUK interaction is essential for the formation of CARMA1 microclusters at the IS. ( a ) AND-Tg T cells expressing a mock-monomeric EGFP or WT, V801P or L815P CARMA1-mEGFP (green) were stained for TCRβ with DyLight 649-conjugated H57 F′ab (red), plated onto an MCC88-103-prepulsed planar bilayer containing I-E k -, ICAM-1- and CD80-GPI and imaged by confocal microscopy at 2 and 30 min after contact. Images of cells before attachment to the bilayer were taken at the equatorial plane of the cells. The percentage of cells forming CARMA1 microclusters at 30 min after contact is shown in b ( n =50). A representative of three independent experiments is shown. Scale bars, 5 μm. Full size image Oncogenic CARMA1 clustering depends on SH3–GUK interactions Oncogenic missense mutations in the C-C domains of CARMA1 in ABC-DLBCLs resulted in a large aggregate formation of mutant proteins in the cytoplasm, correlating with spontaneous activation of the NF-κB pathway [22] . We thus next explored whether SH3–GUK interactions play a role in aggregation and NF-κB activation by oncogenic CARMA1 mutations. Jurkat cells were retrovirally transduced with EGFP-WT CARMA1 or EGFP-CARMA1 L251P, an oncogenic CARMA1 mutant (referred to as Mut2 in the original paper [22] ), with or without V801P or L815P mutations. Cells showing comparable levels of EGFP fluorescence were sorted ( Supplementary Fig. 11c ) and localization of EGFP-CARMA1 molecules was analysed by fluorescence microscopy. As reported previously, over 70% of cells expressing EGFP-CARMA1 L251P had large cytosolic aggregates in the cytoplasm, whereas fewer than 2% of cells expressing EGFP-WT CARMA1 showed aggregate formation ( Fig. 6a,b ). In accord with aggregate formation, cells expressing the L251P mutant produced spontaneous NF-κB reporter activity without any stimulation ( Fig. 6c ) and had greater NF-κB activity than WT-expressing cells after P/I stimulation. Notably, both spontaneous aggregate formation and enhanced NF-κB activity were almost completely lost by V801P or L815P mutation. This indicated that SH3–GUK interactions also control pathogenic signalling clusters formed by oncogenic CARMA1 mutants. 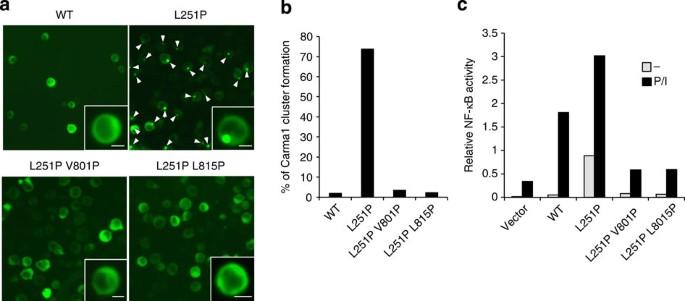Figure 6: Disruption of the SH3–GUK interactions abrogates clustering and NF-kB activation by oncogenic CARMA1. (a,b) Jurkat T cells expressing WT, L251P, L251PV801P or L251PL815P CARMA1-mEGFP (green) were imaged by a fluorescence microscopy (a). Representative images of single cells at a higher magnification are shown in the insets. The arrowheads indicate clusters of CARMA1. Scale bars, 5 μm. The percentage of cells forming CARMA1 clusters is shown inb(n=200). (c) JPM50.6 cells were transfected with plasmids encoding an NF-κB luciferase reporter plasmid (Fireflyluciferase) together with expression plasmids encoding mock, WT, L251P, L251PV801P or L251PL815P CARMA1. Twenty-four hours after transfection, cells were left unstimulated (–) or stimulated with PMA (10 ng ml−1) plus calcium ionophore (1 μM; P/I) for 6 h. Cells were lysed and luciferase activity was determined. All samples were also transfected with constitutively expressedRenillaluciferase to normalize the transfection efficiency. A representative of three independent experiments is shown. Figure 6: Disruption of the SH3–GUK interactions abrogates clustering and NF-kB activation by oncogenic CARMA1. ( a , b ) Jurkat T cells expressing WT, L251P, L251PV801P or L251PL815P CARMA1-mEGFP (green) were imaged by a fluorescence microscopy ( a ). Representative images of single cells at a higher magnification are shown in the insets. The arrowheads indicate clusters of CARMA1. Scale bars, 5 μm. The percentage of cells forming CARMA1 clusters is shown in b ( n =200). ( c ) JPM50.6 cells were transfected with plasmids encoding an NF-κB luciferase reporter plasmid ( Firefly luciferase) together with expression plasmids encoding mock, WT, L251P, L251PV801P or L251PL815P CARMA1. Twenty-four hours after transfection, cells were left unstimulated (–) or stimulated with PMA (10 ng ml −1 ) plus calcium ionophore (1 μM; P/I) for 6 h. Cells were lysed and luciferase activity was determined. All samples were also transfected with constitutively expressed Renilla luciferase to normalize the transfection efficiency. A representative of three independent experiments is shown. Full size image Tanner et al . [31] showed that CARMA1 self-associated through its C-C domains regardless of its activation status. We examined whether V801P or L815P mutations influenced the ability of CARMA1 C-C domains to associate between monomers. We detected the self-association of CARMA1 by immunoprecipitation in a co-expression experiment and observed that this association was dependent on the C-C domain as reported previously [31] ( Supplementary Fig. 13a ). However, the association was not affected by V801P or L815P mutations. In addition, although constitutive CARMA1 aggregation by the L251P mutation in the C-C domain was disrupted by V801P or L815P mutations ( Fig. 6a,b ), these SH3 mutations did not influence interactions between CARMA1 L251P monomers ( Supplementary Fig. 13b ). These findings suggest that the large CARMA1 cluster formation induced by SH3–GUK interactions and the self-association of CARMA1 through the C-C domains appear to be regulated differently. Pomerantz et al . [39] reported that the SH3 and GUK domains, but not the PDZ domain, are indispensable for CARMA1-meditated activation of NF-κB through TCR. Lee et al . [35] reported that the GUK domain binds to PDK1 and that PDK1 silencing affected TCR-induced NF-κB activation. However, the involvement of PDK1 in NF-κB signalling was contradicted in a later study on B cells, where the conditional knockout of PDK1 in chicken DT40 cells did not affect BCR-induced IKK activation [40] . Analysis of the CARMA1 mutation L815P revealed that the SH3 domain of CARMA1 regulates membrane localization of CARMA1, implying the existence of a membrane-associated protein that anchors CARMA1 to the membrane through binding to the SH3 domain [23] . However, currently no candidate protein has been identified. Thus, the molecular mechanisms by which the SH3 and GUK domains of CARMA1 contribute to its function are unclear and some controversy exists between T- and B-cell data. In this study, we identified a novel essential regulation of CARMA1 function via the SH3 and GUK domains that is present both in T and B cells. Previous studies have suggested that the intra- and intermolecular interactions of the SH3–GUK module are conserved among related MAGUK proteins and have a crucial role in regulating the formation and function of signalling complexes at cell–cell junctions in polarized tissues such as epithelia and synapses. Intramolecular interactions of the SH3 domain and the unique-5 (U5) region (which corresponds to the hinge region) with the GUK domain in the rat synapse-associated protein SAP97 interfere with its GUK domain-binding partner GKAP [7] . The SH3 domain of human Dlg (hDlg) binds to the GUK domain of human calcium/calmodulin-dependent serine protein kinase (hCASK) and is required for interaction between hDlg and hCASK [9] . The SH3 and GUK domains of each protein participate in both intra- and intermolecular interactions, although intramolecular one appears to predominate. In addition to that PSD-95 SH3 and GUK domains can self-associate, the PSD-95 GUK domain can bind to the SH3 domain of NE-dlg/SAP102, a MAGUK expressed in neuronal and endocrine tissues, in a Ca 2+ - and calmodulin-dependent manner [41] . The SH3-U5-GUK-U6 domains of the tight junction MAGUK protein ZO-1, which is indispensable for tight junction formation in epithelial cells, are important for the correct localization of ZO-1 as well as the induction of claudin polymerization into tight junction strands [42] . The GUK-U6 domains can bind to the SH3 domain and form intramolecular interactions. Comparison of the crystal structure of the ZO-1 SH3–GUK domain with that of PSD-95 confirmed that the interdependent folding of the SH3 and GUK domains is a conserved feature of these MAGUKs [43] . Importantly, our results demonstrate for the first time that the SH3–GUK interaction-based regulation that is suggested to play a role in MAGUKs in polarized tissues such as epithelia and synapses is also conserved in MAGUK-expressed non-polarized circulating cells, lymphocytes. However, this regulation in lymphocytes also appears to act at a polarized area, the IS formed between T cells and antigen-presenting cells, and likely at the B-cell IS. Oligomerization/clustering of the L-CBM complex is thought to be a key event for activation of the NF-κB pathway. A chromosomal translocation recurrently found in gastric MALT lymphomas, t(11;18)(q21;q21), generates a API2–MALT1 chimera fusion product comprising the N terminus of API2 and the C terminus of MALT1 (ref. 28 ). The fusion product, but neither API2 nor MALT1 alone, potently stimulates NF-κB in the absence of BCL10, likely due to its ability to self-oligomerize without BCL10. Similarly, artificially enforced oligomerization of the MALT1 C terminus triggers NF-κB activation [29] , [30] . A small fraction of recombinant BCL10 forms oligomers in solution and only the oligomerized form can activate IKK in a reconstituted in vitro system [30] . While the primary structures of SH3 and GUK domains are relatively conserved in MAGUKs, the hinge region sequence is not conserved and is unique to each MAGUK. This implies that specific ligands/regulators may act on the hinge region to regulate each MAGUK function. We observed that the flexible hinge region in CARMA1 is required for inhibition of intermolecular SH3 and GUK domain interactions. Thus, as previously proposed for PSD-95 (ref. 25 ), binding of regulators might constrain the flexibility of the hinge region, thereby promoting a switch from intra- to intermolecular assembly of CARMA1, resulting in oligomerization of CARMA1 (L-CBM complex) and cluster formation of the signallosome. However, we have not identified such regulators/regulation and thus still cannot exclude the existence of proteins that might bridge the interaction of CARMA1 monomers through the SH3 and GUK domains. Although we did not find influence of the 801 and 815 mutations on CARMA1 interactions with the key signalling regulators PDK1 and ADAP in co-overexpression studies, it still remains possible that these mutations achieve their deleterious functional effects by perturbing protein–protein interactions with PDK1, ADAP or other proteins in physiological conditions. In this paper, we first demonstrated the functional relationship between the formation of the CARMA1 MCs at the IS and NF-κB signal transduction. Studies have suggested a physical and functional association of CD28-co-stimulation, PKC-θ and L-CBM complex in TCR-induced NF-κB signalling [4] , [23] , [44] , [45] , [46] . CARMA1 is thought to play a central role in the organization of these signalling molecules [4] , and clustering of CARMA1-containing signalling complexes have been suggested to be a key regulation step in activating NF-κB signalling [22] , [29] , [30] , [31] . We recently demonstrated that all of these key proteins involved in NF-κB signalling form MCs similarly in the TCR lo region in cSMAC, segregated from the TCR hi region in a planar lipid bilayer. Importantly, formation of both the CARMA1 and PKC-θ MCs is dependent on CD28 ligand binding [15] , [16] . Thus, these evidences suggest that MCs formed by CARMA1, CD28 and PKC-θ act as signallosomes for NF-κB activation. In conclusion, our results provide the first evidence that intra- and intermolecular interactions between SH3 and GUK domains are conserved in a CARD-MAGUK family protein, CARMA1, in lymphocytes. This interaction regulates not only physiological CARMA1 MC formation at the IS but also oncogenic spontaneous CARMA cluster formation, essential for activation of the NF-κB pathway. Our results indicate that therapeutic inhibition of these interactions might be particularly effective to attenuate ABC-DLBCLs harbouring oncogenic CARMA1 mutations. Cells and mice JGFP1 and JPM50.6 cells were generated previously as described [32] and provided by X. Lin (University of Texas M.D. Anderson Cancer Center). Carma1 –/– mice were generated previously as described [37] . AND-Tg mice on Rag2 –/– background were provided by R.N. Germain (National Institutes of Health, NIH). C57BL/6J mice were purchased from Japan Clea or Kyudo. Mice were maintained in our animal facility and treated in accordance with the ethical guidelines of Saga University. Generation of L815P knock-in mouse To generate the CARMA1 L815P knock-in ( Carma1 L815P ) mouse, the CARMA1 gene was isolated from genomic DNA extracted from embryonic stem (ES) cells (R1) by PCR. A genomic fragment containing exon 18 of IRAK-4 was cloned and point mutation resulting in the L815P conversion in the SH3 domain was introduced by a site-directed mutagenesis. In the targeting vector, a neomycin-resistance gene cassette (neo) flanked with two loxP sites and a diphtheria toxin A gene cassette (for negative selection) driven by a PGK promoter were inserted into the genomic fragment. After the targeting vector was transfected into ES cells, G418-resistant colonies were selected, screened by PCR and further confirmed by Southern blotting. Three clones with homologous recombination were injected into blastocysts from C57BL/6 females. The obtained chimeric males were crossed with C57BL/6 females, and the F1 generations obtained with mutated CARMA1 were crossed with CAG-Cre transgenic mice to excise the neo cassette. The CAG-Cre transgene was removed from Carma1 L815P heterozygous mice without a neo cassette by crossing the mice with C57BL/6 mice, then intercrossing to obtain Carma1 L815P homozygous mice. The Carma1 L815P mice were backcrossed for at least five generations onto the C57BL/6J background. Sequence alignment and molecular modelling The sequences of human CARMA1 and human CARMA3 were obtained from NCBI server (accession: NP_115791.3 and NP_055365.2, respectively). The crystal structure of rat PSD-95 was obtained from the Protein Data Bank (PDB ID: 1kjw) as a template for generating a homology model. 3D structures of SH3 and GUK domains of CARMA1 or CARMA3 were modelled using MODELLER 9v8 software with default parameters [47] . Sequences of SH3–GUK modules between human CARMA1 or human CARMA3 and rat PSD-95 were aligned using CLUSTALW [48] , and the resulting alignments were used for homology modelling. In total, 50 structures were generated for each domain from CARMA1 or CARMA3 using the aa sequence 430–503 for the SH3 domain and the aa sequence 521–724 for the GUK domain of PSD-95. The stereochemical qualities of the generated structures were estimated using PROCHECK software [49] , and the structure with highest G-factor value was selected for further analysis. Supplementary Figs 2b and 3b were produced with UCSF Chimera (RBVI). Antibodies and reagents Antibodies specific for Erk (9102) (1:1,000), phospho-Erk (9101) (1:1,000), p38 (9212) (1:1,000), phospho-p38 (9102) (1:1,000), Jnk (9258) (1:1,000), phospho-Jnk (9251) (1:1,000), I-κBα (9242) (1:1,000) and phospho-I-κBα (2859) (1:1,000) were from Cell Signaling Technology; antibodies specific for CD4 (L3T4) (1:200), CD8 (53-6.7)v, B220 (RA3-6B2) (1:200), IgM (II/41) (1:200), IgD (11–26) (1:200), CD5 (53-7.3) (1:200), CD21 (eBio4E3) (1:200), CD23 (B3B4) (1:200), FoxP3 (FJK-16a) (1:100), mouse CD3ε (145-2C11) (1 or 10 μg ml −1 ), mouse CD28 (37–51) (1 or 10 μg ml −1 ), human CD3ε (OKT-3) (1, 3 or 10 μg ml −1 ) and human CD28 (CD28.2) (1 μg ml −1 ) were from eBioscience; anti-actin antibody (sc-8432) (1:1,000) was from Santa Cruz Biotechnology; F(ab′)2 fragment of anti-mouse IgM (715-006-020) (2, 6 or 20 μg ml −1 ), goat anti-hamster IgG (H+L) (127-005-099) (10 μg ml −1 ) and TRITC-conjugated anti-rabbit IgG (H+L) (211-025-109) (1:1,000) were from Jackson ImmunoResearch; Rabbit anti-CARMA1 COOH-terminus polyclonal antibody was generated as previously described [37] ; PMA, ionomycin (calcium ionophore A231877), LPS (from O111:B4, L3024), anti-Flag antibody (M2) (1:1,000), anti-Myc (9E10) (1:1,000) antibodies and fluorescein isothiocyanate (FITC)-conjugated cholera toxin β-subunit (CTX-B, C1655) were from Sigma; anti-rat CD2 antibody (CL034) (1:500) was from Cedarlane; and 4,6-diamidino-2-phenylindole (DAPI) was from Molecular Probes. Plasmids and transfectants Myc- and Flag-epitope-tagged human CARMA1 and its mutants were generated by PCR and subcloned into pcDNA3.1 (Invitrogen) or the retroviral vector pMX-IRES-rCD2 (provided by M. Kubo, RIKEN Research Center for Allergy and Immunology, Yokohama, Japan). CARMA1 point mutants (V801P, L815P, L251P, L251PV801P and L251PL815P) were generated using site-directed mutagenesis and confirmed by sequencing analysis. The aa sequences corresponding to the following CARMA1 constructs are in parentheses: Flag-ΔPDZ (1–666, 768–1,154), Flag-ΔSH3 (1–767, 902–1,154), Flag-ΔGUK (1–959), Flag-ΔGUKΔSH3 (1–767), Flag-ΔHinge (1–836, 960–1,154), Flag-ΔHinge+6Gly (1–836–(6 × Gly)–960–1,154), Myc-GUK (902–1,154) and Myc-GUKΔβF (902–1,142). Plasma membrane-targeted CARMA1 constructs (MP-WT, MP-CARMA1, MP-V801P, MP-L815P) containing the MP motif of the Lck tyrosine kinase (MGCGCSSHPE) [34] at the N terminus were generated by PCR using cDNA encoding WT, V801P and L815P CARMA1 as template DNAs. Retrovirus-mediated gene transfer to Jurkat or JPM50.6 cells was performed as previously described by using the retroviral vectors, pMX or pMX-IRES-rCD2 (ref. 50 ). At days 1 and 2, tenfold-concentrated retrovirus supernatant was added, followed by centrifugation at 800 g for 1 h. Then, 4 days after infection, EGFP + cells (for transduction of mEGFP-tagged proteins) or rCD2 + cells (for transduction of pMX-IRES-rCD2 constructs) were sorted using FACSAria (BD) and were used for assays. Retroviral transduction of AND-Tg CD4 + T cells with expression constructs for mEGFP-tagged CARMA1 and its mutants was performed as previously described [16] . At day 3 or later post viral transfection, EGFP-positive cells were sorted with FACSAria (BD) to obtain populations with homogenous fluorescence intensity. Cells were maintained for 5–14 days in RPMI1640 medium containing 10% fetal calf serum supplemented with recombinant IL-2. For co-immunoprecipitation assays, 1 μg of various Flag/Myc-tagged constructs was transfected into 1 × 10 5 of HEK293 cells plated on a six-well culture dish by lipofection using Lipofectamine LTX (Invitrogen) according to the manufacturer’s instructions. After 24 h incubation, proteins were immunoprecipitated with anti-Flag antibody and protein A-agarose (Roche Applied Science). Samples were washed four times with lysis buffer (50 mM HEPES, pH 7.4, 1 mM EDTA, 250 mM NaCl and 1% Nonidet P-40) and eluted with SDS loading buffer. The eluted samples were subjected to SDS–PAGE and western blotting with anti-Myc antibody. Full scans of western blots in the main figures are shown in Supplementary Fig. 14 . Yeast two-hybrid screening The two-hybrid analysis was performed by the Hitachi Life Science Group using an automated process with ProNet technology for large-scale identification of protein–protein interactions that are based on nuclear yeast two-hybrid methodologies (Myriad Genetics) as described previously [51] . Mouse spleen was used to prepare prey libraries. Baits were mated with prey, and selection was based on the drop-out media (-Trp, -Leu, -His, -Ade) plates. Interactions between bait and prey molecules were identified using His- and Ade- selections. Plasmids isolated were retransformed into yeast, and interactions were confirmed by galactosidase assays. The specificity of the prey was investigated in a separate false-positive test where the prey was tested against a mixture of several heterologous baits. The identities of the prey were determined by DNA sequencing. Planar bilayers and microscopic imaging The purification of GPI-anchored proteins was described previously [52] . Briefly, GPI-anchored proteins were incorporated into dioleoyl phosphatidylcholine liposomes (DOPC; Avanti Polar Lipids) and incubated between coverslips in a flow cell chamber (Bioptechs). The expression level of each GPI-anchored protein was quantified as previously described [16] and adjusted as follows: I-E k , 250 molecules μ −1 m −2 ; ICAM-1, 100 μ −1 m −2 ; and CD80, 150 μ −1 m −2 . The planar bilayers were loaded with 10 μM MCC88-103 in citrate buffer (pH 4.5) for 24 h at 37 °C, blocked with 5% non-fat dried milk in phosphate-buffered saline (PBS) for 1 h at 37 °C and left to stand in the assay medium (HEPES-buffered saline) containing 1% fetal calf serum, 2 mM MgCl 2 and 1 mM CaCl 2 . AND-Tg T cells expressing WT, V801P or L815P CARMA1 tagged with mEGFP and stained with fluorescent-labelled H57 Fab′ were allowed to settle on the bilayer and visualized using confocal microscopy (Leica, SP5). Lymphocyte preparation Whole T cells from lymph nodes or spleen were purified with magnetic-activated cell sorting (Miltenyi Biotec) to remove B220 + , NK1.1 + , Mac-1 + and Gr-1 + cells. The CD3 + purity was >95% by fluorescence-activated cell sorting (FACS). Splenic B cells were purified using magnetic-activated cell sorting to remove CD3 + , NK1.1 + , Mac-1 + and Gr-1 + cells, and B220 + purity was >95% by FACS. Flow cytometry and immunocytochemistry For flow cytometry, single-cell suspensions of thymus, lymph node, bone marrow, spleen and peritoneal exudates were stained with FITC-, phycoerythrin- or allophycocyanin (APC)-conjugated antibodies, such as CD3ε, CD4, CD8, FoxP3, B220, IgM, IgD, CD5, CD21 and CD23. For intracellular staining of Foxp3, the Foxp3-Staining Buffer Set (eBioscience) was used according to the manufacturer’s instructions. The stained cells were analysed with a FACSCalibur flow cytometer (Becton Dickinson) using CellQuest software (BD Biosciences). For immunocytochemistry of JPM50.6 cells reconstituted with CARMA1 and its mutants, cells were stained with FITC-conjugated CTX-B (8 μg ml −1 ) for 10 min on ice and then fixed with 4% paraformaldehyde for 10 min at room temperature. Cells were permeabilized with PBS containing 1% bovine serum albumin and 0.05% Triton X for 1 min and stained with rabbit anti-CARMA1 polyclonal antibody followed by TRITC-conjugated anti-rabbit IgG (5 μg ml −1 ) and DAPI (5 μg ml −1 ) in PBS containing 1% bovine serum albumin for 30 min at room temperature. BZ8000 (Keyence) was used for deconvoluted fluorescence imaging. Antigen receptor signalling and EMSA assays For antigen receptor signalling assays, T cells were stimulated either with hamster anti-CD3ε plus hamster anti-CD28 followed by crosslinking with anti-hamster IgG (H+L), or with PMA plus calcium ionophore (P/I). B cells were stimulated with anti-mouse IgM F(ab′) 2 or P/I. After incubation at 37 °C for various time periods, cells were lysed in ice-cold lysis buffer (50 mM Tris-HCl (pH 8.0), 150 mM NaCl, 1.0% Triton X-100, 20 mM EDTA, 1 mM Na 3 VO 4 , 1 mM NaF and protease inhibitors) and subjected to western blotting using antibodies against phospho-ERK1/2, ERK1/2, phospho-p38-MAPK, p38-MAPK, phospho-JNK, JNK, phospho-IκBα, IκBα and actin (C-2, Santa Cruz Biotechnology). For electromobility shift assays, nuclear extracts were prepared according to previously described protocols [53] . In brief, protein extracts (4 μg) were incubated in 20 μl binding buffer with DIG-end-labelled, double-stranded oligonucleotide NF-κB probe (5′- ATCAGGGACTTTCCGCTGGGGACTTTCCG -3′) and fractionated on a 5% polyacrylamide gel. The NF-κB binding buffer was 5 mM HEPES (pH 7.8), 50 mM KCl, 0.5 mM dithiothreitol, 2 μg poly (dI-dC) and 10% glycerol. Measurement of serum immunoglobulin levels Basal levels of Ig isotypes were analysed by ELISA (enzyme-linked immunosorbent assay) on serially diluted serum samples using anti-mouse IgG1, IgG2a, IgG2b, IgG3, IgA or IgM antibodies (Southern Biotechnology Associates) according to the manufacturer’s directions. Ex vivo functional analysis of T and B cells For proliferation assays, T cells were stimulated with plate-bound anti-CD3ε alone or anti-CD3ε plus anti-CD28 or with P/I. B cells were stimulated with anti-IgM F(ab′) 2 fragment or LPS. The culture after 2 days was pulsed with 1 μCi of [ 3 H]-thymidine (Amersham) for 8 h and harvested. [ 3 H]-thymidine incorporation was measured with Microbeta (PerkinElmer) or Matrix 96 (Packard). For the cytokine production assay, the culture supernatants of T cells were assayed in triplicate for the production of IL-2 by ELISA (R&D Systems). Reporter assays for NF-κB activity JPM50.6 cells (5 × 10 5 ) in six-well plates were transfected with 1.5 μg of the NF-κB-dependent luciferase (firefly) reporter plasmid pBXIV-Luc (provided by Dr W.C. Yeh, Amgen) and 0.2 μg of the HSV-TK promoter-regulated Renilla luciferase reporter plasmid pRL-TK (Promega) together with 0.3 μg expression vectors for CARMA1 and its mutants or mock vector (pcDNA3.1) using Lipofectamine LTX (Invitrogen) according to the manufacturer’s instructions. After 16 h incubation, cells were left unstimulated or stimulated with PMA (10 ng ml −1 ) plus anti-CD28 (3 μg ml −1 ) or Raji B cells (2.5 × 10 5 ) pulsed with 10 ng ml −1 of SEE (Toxin Technology, Sarasota, FL) for 6 h. Luciferase activity in the cell lysate was determined using the Dual-Luciferase kit (Promega). Subcellular fractionation Cytosolic and membrane fractions were prepared as described [54] . Briefly, cells were lysed with subcellular fractionation buffer (250 mM sucrose, 20 mM HEPES (pH 7.4), 10 mM KCl, 1.5 mM MgCl 2 , 1 mM EDTA, 1 mM EGTA, 1 mM DTT and protease inhibitors), and nuclear extracts were removed by centrifugation at 720 g for 5 min and centrifuged again at 10,000 g for 5 min. The supernatants were then ultracentrifuged at 100,000 g for 1 h. The supernatants were collected as cytosolic fractions, whereas the pellets were collected as membrane fractions. Preparation of recombinant proteins Recombinant Flag-SH3, Flag-SH3 V801P, Flag-SH3 L815P and His-GUK proteins were produced using the FreeStyle 293 Expression system (Invitrogen). Briefly, fragments encoding Flag-SH3, Flag-SH3 V801P, Flag-SH3 L815P and His-GUK were cloned into a pcDNA3.1 expression vector (Invitrogen) and were then transiently transfected into the FreeStyle 293-F cells (Invitrogen). After 3 days, the transfected cells were collected, lysed and centrifuged at 12,000 g for 10 min. Recombinant proteins were purified from the supernatants using the FLAG M Purification kit (Sigma) for Flag-tagged proteins or the His GraviTrap (GE Healthcare) for His-tagged proteins according to the manufacturer’s instructions. Statistical analysis Statistical differences between groups were analysed using the Student’s t -test. Differences with P values <0.05 were considered significant. How to cite this article: Hara, H. et al . Clustering of CARMA1 through SH3–GUK domain interactions is required for its activation of NF-κB signalling. Nat. Commun. 6:5555 doi: 10.1038/ncomms6555 (2015).